Enantioselective total syntheses of (+)-stemofoline and three congeners based on a biogenetic hypothesis The powerful insecticidal and multi-drug-resistance-reversing activities displayed by the stemofoline group of alkaloids render them promising lead structures for further development as commercial agents in agriculture and medicine. However, concise, enantioselective total syntheses of stemofoline alkaloids remain a formidable challenge due to their structural complexity. We disclose herein the enantioselective total syntheses of four stemofoline alkaloids, including (+)-stemofoline, (+)-isostemofoline, (+)-stemoburkilline, and (+)-(11 S ,12 R )-dihydrostemofoline, in just 19 steps. Our strategy relies on a biogenetic hypothesis, which postulates that stemoburkilline and dihydrostemofolines are biogenetic precursors of stemofoline and isostemofoline. Other highlights of our approach are the use of Horner–Wadsworth–Emmons reaction to connect the two segments of the molecule, an improved protocol allowing gram-scale access to the tetracyclic cage-type core, and a Cu-catalyzed direct and versatile nucleophilic alkylation reaction on an anti-Bredt iminium ion. The synthetic techniques that we developed could also be extended to the preparation of other Stemona alkaloids. Nature continues to serve as an invaluable source for the development of pharmaceutical drugs [1] , agrochemical agents [2] , and biomedical probes [3] . In this context, efficient total synthesis of these bioactive natural products is of crucial importance [4] . With significant advances in synthetic methodologies and strategies, many artful instances of total synthesis have been documented in the last few decades [4] . However, most of these reported studies involved only one target molecule [5] . Considering the huge number of biologically interesting natural products, there is clearly unmet need in developing novel synthetic strategies that can branch out toward multiple target compounds. In recent years, multi-target-oriented synthetic approaches, such as unified strategy [6] , [7] , [8] , [9] , collective synthesis [10] , [11] , and diversity-oriented synthesis [12] , have emerged as a frontier. It should be noted that many of these methods are biomimetic or bioinspired in that they rely on known biogenetic routes or hypotheses. But for those natural products whose biogenetic pathways are unknown or have not been investigated in detail, it is necessary to develop biogenetic hypotheses [13] , [14] . The Stemona alkaloids are a class of structurally diverse natural products that act as the principle active constituents in Stemona plants (Stemonaceae) [15] , [16] , [17] , [18] , [19] , [20] . Known as “Bai Bu” in traditional Chinese medicine, Stemona plants have been used in East Asia for thousands of years as insecticides and anti-cough agents [15] , [16] , [19] , [20] . To date, more than 215 Stemona alkaloids have been isolated [15] , classified by Pilli [19] , [20] into eight structural groups (see Supplementary Fig. 1 ). The attractive bioactivities [15] , [16] and unique polycyclic structures of these alkaloids have led to intense phytochemical, synthetic, and biomedical investigations, and many innovative total syntheses have been achieved [16] , [18] , [19] , [20] , [21] , [22] , [23] , [24] . The stemofoline group of alkaloids (Fig. 1 ) are a highly versatile set of compounds that represent promising lead structures for agricultural and medicinal applications [15] , [16] . Stemofoline ( 1 ), the parent member of the stemofoline group, was isolated first from Stemona japonica by Irie and coworkers in 1970 [25] , and then from several other Stemona species. Its structure, including the absolute configuration, was determined by single-crystal X-ray crystallographic analysis [25] . To date, more than twenty members of the stemofoline group have been isolated and structurally determined, including isostemofoline ( 2 ) [26] , didehydrostemofoline ( 3 ) [27] , [28] , isodidehydrostemofoline ( 4 ) [27] , methoxystemofoline ( 5 , suggested structure) [29] , methylstemofoline ( 6 ) [30] , stemoburkilline ( 7 ) [31] , [32] , and (11 S ,12 R )-dihydrostemofoline ( 8 ) [31] (Fig. 1 ). The high insecticidal activity [33] of stemofoline ( 1 ) was first reported in 1978, according to which the compound acts as a potent agonist of the insect nicotinic acetylcholine receptors (nAChR) (EC 50 = 1.7 nM) and is associated with acetylcholinesterase (AChE) inhibition [15] . Ye and coworkers have established that the cage-type moiety of stemofoline is pivotal to its insecticidal activity [26] . Notably, by using stemofoline ( 1 ) as a lead, synthetic cyanotropanes have been developed as a class of commercial insecticides [2] . Moreover, stemofoline ( 1 ) has been found to alleviate inflammation [34] and reverse multidrug resistance of certain types of cancer [15] , [35] , [36] , [37] . Indeed, it has been shown that stemofoline ( 1 ) increases the sensitivity of patients toward anticancer drugs such as vinblastine, paclitaxel, and doxorubicin [15] , [35] . Once again, this desirable properties can be attributed to the core cage structure with nonpolar side chains [35] . Fig. 1: Structures of representative stemofoline alkaloids. a Z -Series: (+)-stemofoline ( 1 ); (+)-didehydrostemofoline ( 3 ); (+)-methylstemofoline ( 6 ). b E -Series: (+)-isostemofoline ( 2 ); (+)-isodidehydrostemofoline ( 4 ); (+)-methoxystemofoline ( 5 ) (revised structure). c 11,12-Dihydro series: (+)-stemoburkilline ( 7 ); (+)-(11 S , 12 R )-dihydrostemofoline ( 8 ). Full size image Much efforts have been devoted to the synthesis of stemofoline alkaloids. Starting from stemofoline [38] and (11 Z )-1′,2′-didehydrostemofoline [39] , [40] , several semisynthetic stemofoline alkaloids and analogues have been prepared and screened by Ye et al. and Pyne et al., respectively. Although tremendous efforts have been devoted to the total synthesis of these alkaloids [41] , [42] , [43] , [44] , [45] , [46] , [47] , successful examples remain rare, including racemic total syntheses of isostemofoline ( 2 ) by Kende [48] and didehydrostemofoline (asparagamine A, 3 ) and isodidehydrostemofoline ( 4 ) by Overman [49] , and enantioselective formal total syntheses of didehydrostemofoline and isodidehydrostemofoline by Martin [50] . Notably, although stemofoline ( 1 ) displays remarkable bioactivities, and has proven to be a promising lead for the development of insecticide and anticancer agents, its total synthesis has not yet been achieved. As a part of our efforts to achieve efficient total synthesis of structurally complex, enantiopure alkaloids [51] , we have been focused in the last decade on developing versatile methodologies for the direct transformation of amides [52] , [53] . We have recently reported a method for the construction of tropinone ring systems [54] and applied it to the total synthesis of (+)-methoxystemofoline ( 5 ) [55] . We disclose herein biogenetic hypothesis-based syntheses of (+)-stemofoline ( 1 ), (+)-isostemofoline ( 2 ), (+)-stemoburkilline ( 7 ), (11 S ,12 R )-dihydrostemofoline ( 8 ), and diastereomer 9 . Biogenetic hypothesis Structurally, stemofoline alkaloids consisted of a tetronate moiety connected through an ene diether (C11–C12) to a cage-like aza-pentacyclic ring system. Both the enantioselective construction of the cage-like aza-pentacyclic ring system [56] and the stereoselective formation of the ene diether moiety are challenging [48] , [49] , [55] . Indeed, our previous total synthesis was lengthy and contained several steps of reaction with low chemo-, regio-, and/or diastereoselectivity [55] . In addition, the stemofoline alkaloids display great variation in the oxidation state and connectivity at C11, the stereochemistry of the ene diether connector, and substitution at the bridgehead carbon C3. Taking these factors into consideration, we wanted to develop a concise, versatile synthetic strategy. Although a bioinspired approach is highly desirable [57] , and indeed there are already several hypotheses on the origin of the central building blocks in Stemona alkaloids [15] , [16] , [17] , [28] , the basic biogenetic steps in the formation of Stemona alkaloids remain unknown [15] . In the search for a biogenetic relationship between the stemofoline group of alkaloids, we have noted that isostemofoline ( 2 ) [26] , stemoburkilline ( 7 ), and (11 S ,12 R )-dihydrostemofoline ( 8 ) [31] , [32] were congeners of stemofoline ( 1 ), and Pyne et al. also observed that (11 S ,12 S )-dihydrostemofoline ( 9 ) (Fig. 2a ) could be converted into a mixture of stemoburkilline ( 7 ) and (11 S ,12 R )-dihydrostemofoline ( 8 ) upon treatment with DBU [32] . Moreover, Ye and coworkers [26] have reported the co-existence of stemofoline ( 1 ) and isostemofoline ( 2 ), the latter as a minor congener, in S. japonica , whereas Jiwajinda et a l. has detected equal amounts of 11 Z -didehydrostemofoline ( 3 ) and 11 E -didehydrostemofoline ( 4 ) in S. collinsae [27] . Combining these findings with ours, we hypothesized that the known compounds stemoburkilline ( 7 ) and (11 S ,12 R )-dihydrostemofoline ( 8 ), and possibly the unknown compound (11 S ,12 S )-dihydrostemofoline ( 9 ), are plausible biogenetic precursors of stemofoline ( 1 ) and isostemofoline ( 2 ) (Fig. 2a ). Fig. 2: Our biogenetic hypothesis and retrosynthetic analysis of stemofoline alkaloids. a Our biogenetic hypothesis. b Retrosynthetic analysis based on our biogenetic hypothesis. Full size image Retrosynthetic analysis Guided by our biogenetic hypothesis (Fig. 2a ), we conducted a retrosynthetic analysis of stemofoline ( 1 ) as depicted in Fig. 2b . The ( Z )-5-(dihydrofuran-2(3 H )-ylidene)-4-methoxy-3-methylfuran-2(5 H )-one [( Z )-ene diether moiety could be constructed through C–H oxygenation of stemoburkilline ( 7 ). The functionalized C11–C12 alkene moiety in 7 could be assembled through Horner–Wadsworth–Emmons-type reaction of diethyl (3-methoxy-4-methyl-5-oxo-2,5-dihydrofuran-2-yl)phosphonate ( 10 ) with the pentacyclic cage-type hemiacetal 11 . Other key issues to be addressed were: (1) the O -debenzylation of 13 triggering double cyclization, (2) the direct, chemo-, regio-, and diastereoselective methylation at C10 to build a chiral canter, and (3) direct installation at C3 a butyl group or other alkyl groups needed for the synthesis of other stemofoline alkaloids and analogues. Syntheses of stemoburkilline (7), its congeners 8, and 9 To implement our strategy, we first developed an improved five-step protocol to furnish the tropinone building block 16 on a multi-gram scale (Fig. 3 ). To this end, commercially available α-benzyloxy-γ-lactone ( S )- 18 was treated with O -silylated β-aminoethanol 19 in methanol at room temperature for 2–3 days, which afforded γ-hydroxyamide 20 in 90% yield. Swern oxidation of 20 generated a diastereomeric mixture of hemiaminals, which was then subjected without purification to NaH-mediated Horner–Wadsworth–Emmons reaction with dimethyl (2-oxopropyl)phosphonate ( 21 ) followed by cyclization to produce the desired cis -ketolactam 17 in 60% yield (over two steps), along with the trans -diastereomer in 21% yield. Conversion of 17 to bromo-tropinone building block 16 was achieved in 78% yield via a two-step keto-lactam cyclization-bromination cascade (TMSOTf, Et 3 N, CH 2 Cl 2 , 0 °C; Tf 2 O, DTBMP, ZnBr 2 , CH 2 Cl 2 , −78 °C to rt) that we previously developed [54] . Fig. 3: Enantioselective synthesis of the tropinone building block 16. Reagents and conditions: a 19 , MeOH, rt, 3 d, 90%; b (COCl) 2 , DMSO, Et 3 N, CH 2 Cl 2 , −78 °C; c NaH, 21 , THF, 0 °C to reflux, 60% (for 2 steps); d TMSOTf, Et 3 N, CH 2 Cl 2 , 0 °C, e Tf 2 O, DTBMP, ZnBr 2 , CH 2 Cl 2 , −78 °C to rt, 78% (for 2 steps from cis - 17 ). Full size image We next focused on the development of a direct and versatile method for the installation of an n -butyl group on the bridgehead carbon of 16 . In our previous strategy [55] , three steps were required to introduce the 4-methoxybutyl group. A survey of literatures indicated that the bridgehead nitrogen in similar but simpler ring systems, such as 1-chloro-9-methyl-9-azabicyclo[3.3.l]nonane, enhances the rate of solvolysis dramatically [58] . However, attempted direct alkylation of a similar α-chloroamine with organolithium or Grignard reagent produced disappointing results [59] , [60] . Encouragingly, Kibayashi and coworkers have reported that bridged tricyclic N , O -acetals can be alkylated using Grignard reagents in the presence of Et 2 AlCl through S N 1 reaction on bridgehead anti-Bredt iminium ion intermediates [60] , [61] . In light of these precedents, we opted to explore whether metal-catalyzed direct alkylation of 3-bromotropinone building block 16 with Grignard reagents was feasible. After extensive screening (cf. 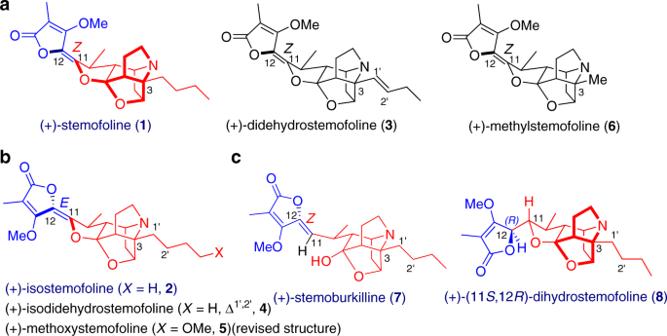Fig. 1: Structures of representative stemofoline alkaloids. aZ-Series: (+)-stemofoline (1); (+)-didehydrostemofoline (3); (+)-methylstemofoline (6).bE-Series: (+)-isostemofoline (2); (+)-isodidehydrostemofoline (4); (+)-methoxystemofoline (5) (revised structure).c11,12-Dihydro series: (+)-stemoburkilline (7); (+)-(11S, 12R)-dihydrostemofoline (8). Table 1 ), we achieved gram-scale coupling of 16 with n -butyl magnesium bromide in THF to afford the desired butylated product 15 in 81% yield, with CuCl 2 as a catalyst, TMEDA ( N , N , N ′, N ′-tetramethylethylenediamine) as ligand and LiOMe as additive (Table 1 , entry 12). According to the precedent set by Kibayashi, it is possible that the alkylation reaction involves an S N 1 mechanism via the intermediacy of anti-Bredt bridgehead iminium ion A . Significantly, the method can be extended to other Grignard reagents, thereby allowing the introduction of other desired simple or functionalized alkyl groups at C3. In this manner, alkylated products 15a – 15d (Fig. 4 ) could be prepared directly from 16 in good yields (75–85%). Table 1 Screening of reaction conditions for the butylation of 16 with n -BuM. Full size table Fig. 4: Direct alkylation of 16 with Grignard reagents. Reagents and conditions: a CuCl 2 , TMEDA, LiOMe, RMgBr, THF, rt, 30 min. Full size image To construct compound 14 , which contains a tricyclic core with an ester-enone moiety (Fig. 5 ), tropinone 15 was successively treated with LDA and ethyl glyoxalate ( 22 ) to yield aldol adducts 23-1 and 23-2 in 71% yield with a diastereomeric ratio of 1.1:1, along with regioisomer 23a in 15% yield. The lack of diastereoselectivity was of no consequence as dehydration of 23-1 and 23-2 afforded the desired enone 24 as a single isomer in 72% yield. NOESY studies indicated that 24 adopted an E configuration (see Supplementary Fig. 3 ). From these experimental results, we deduced that the structures of two diastereomers 23-1 and 23-2 have the stereochemistries shown in Fig. 5 . Fig. 5: Synthesis of the pentacyclic lactone 12. Reagents and conditions: a LDA, ethyl glyoxalate ( 22 ), −78 °C, 1.5 h, 71% for 23 and 15% for 23a ; ( b ) CDI, i -Pr 2 NEt, DMAP, CH 2 Cl 2 , 0 °C to rt, 4 h, 72%; c p -TsOH, acetone, 50 °C, 30 min, 96%; d CBr 4 , PPh 3 , CH 2 Cl 2 , 0 °C, 30 min, 95%; e EtONa, THF, 0 °C, 20 min, 95%; f MeLi, DMPU, Et 2 O, −40 °C, 20 min, 86%; g Pd/C, H 2 , EtOH, rt, 2 d, 87%; h p -TsOH, toluene, 85 °C, 2 h, 93% (83% for two steps from 13 without further purification). Full size image Desilylation of 24 with p -TsOH, followed by bromination of the resultant alcohol 25 , furnished tropinone halide 26 in an overall yield of 91.2% (for 2 steps; Fig. 5 ). Exposure of 26 to EtONa in THF resulted in the formation of tricyclic enone 14 in excellent yield (95%). Another key step for our strategy resided in the regio- and diastereoselective methylation at C10. To our delight, the intended conjugate addition was achieved by treating 14 with MeLi-DMPU in diethyl ether [62] , leading to 13 as a single regio- and diastereomer in 86% yield. Pd/C catalyzed O -debenzylation of 13 in ethanol was accompanied by tandem lactolization, which furnished the cage-like core structure 27 directly as a single diastereomer in 87% yield. Exposing 27 to p -TsOH in toluene produced the key pentacyclic lactone 12 in 93% yield. Importantly, neither the hydrogenation nor lactonization step required purification to yield 12 of sufficient purity for further reactions. The stereochemistry of 12 was determined by NOESY experiments (see Supplementary Fig. 6 ), which confirmed that the addition of MeLi to 14 was instrumental in creating the two vicinal chiral centers at C9 and C10. After 12 was synthesized, it was reduced with DIBAL-H to afford hemiacetal 11 as an inseparable diastereomeric mixture in 78% yield (Fig. 6 ). Once again, the lack of diastereoselectivity did not matter because treatment of 11 with potassium t -butoxide and diethyl (3-methoxy-4-methyl-5-oxo-2,5-dihydrofuran-2-yl)phosphonate ( 10 ), prepared in one-pot from γ-bromotetronate [63] , resulted in the formation of stemoburkilline ( 7 ), (11 S ,12 R )-dihydrostemofoline ( 8 ), and the diastereomeric (11 S ,12 S )-dihydrostemofoline ( 9 ), in 27%, 24%, and 33% yield, respectively (combined yield: 84%). 1 H and 13 C nuclear magnetic resonance (NMR) and polarimetric data of 7 – 9 were largely consistent with previously reported values (see Supplementary Tables 5 – 10 ) [31] , [32] . Fig. 6: Completion of the total syntheses of stemoburkilline (7), (11 S ,12 R )-dihydrostemofoline (8), and (11 S ,12 S )-dihydrostemofoline (9). Reagents and conditions: a DIBAL-H, CH 2 Cl 2 , −78 °C, 30 min, 78%; b t -BuOK, 10 , THF, 0 °C, 30 min, 84% (27% for 7 ; 24% for 8 ; 33% for 9 ); c LHDMS, THF, −78 °C, 1 h, 98%. Full size image Given that the treatment of (11 S ,12 S )-dihydrostemofoline ( 9 ) with DBU yielded a tautomeric mixture of 9 , (11 S ,12 R )-dihydrostemofoline ( 8 ), and stemoburkilline ( 7 ) in a ratio of 39:37:24 [32] , we speculated that stemoburkilline ( 7 ) could be a kinetic tautomer and that, under kinetic conditions, it would be possible to selectively convert both 8 and 9 into 7 . Indeed, treatment of a mixture of 8 and 9 with LHMDS resulted in the formation of stemoburkilline ( 7 ) in 98% yield (Fig. 6 ). Total syntheses of stemofoline (1) and isostemofoline (2) To complete the total synthesis of stemofoline, a one-step Wacker-type reaction of stemoburkilline ( 7 ) was explored. Unfortunately, none of the reaction conditions (Na 2 PdCl 4 , TBHP [64] , [65] ; PdCl 2 , CuCl, O 2 [66] , [67] ; Pd(TFA) 2 , IMes [68] ) (see Supplementary Table 1 ) that we tested yielded the desired final product stemofoline ( 1 ). In each instance, a complex mixture of by-products, decomposition of the starting material, or lack of any major reaction whatsoever, was observed. Next, we envisioned a two-step dehydrogenation of 8 and 9 consisting of introduction of a leaving group at C12 followed elimination. 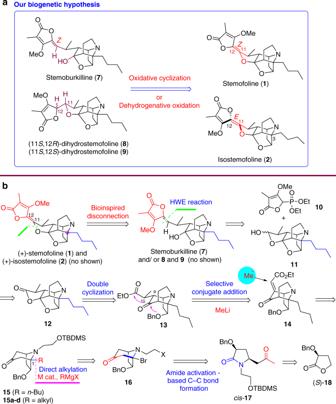Fig. 2: Our biogenetic hypothesis and retrosynthetic analysis of stemofoline alkaloids. aOur biogenetic hypothesis.bRetrosynthetic analysis based on our biogenetic hypothesis. However, oxygenation with IBX/DMSO or DBU/O 2 , halogenation with NIS/NBS, or methylsulfidation with MeSSMe, are all found to be disappointingly inadequate (see Supplementary Table 2 ). 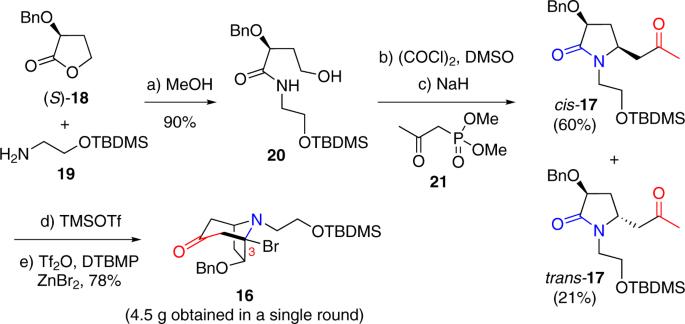Fig. 3: Enantioselective synthesis of the tropinone building block 16. Reagents and conditions:a19, MeOH, rt, 3 d, 90%;b(COCl)2, DMSO, Et3N, CH2Cl2, −78 °C;cNaH,21, THF, 0 °C to reflux, 60% (for 2 steps);dTMSOTf, Et3N, CH2Cl2, 0 °C,eTf2O, DTBMP, ZnBr2, CH2Cl2, −78 °C to rt, 78% (for 2 steps fromcis-17). Attempted conversion of 8 and 9 to 1 (see Supplementary Table 3 ) through cyclization to form 29 followed by oxidation was also unsuccesful because treating a mixture of 8 and 9 with LHMDS and TMSCl resulted in no cyclization and exclusive formation of an O -TMS derivative 30 in 93% yield (Fig. 7a ). We then turned our attention to the electrophilic cyclization of 7 . However, 7 apparently showed no reaction with NIS and was thus mostly recovered (>95%), regardless of whether CH 2 Cl 2 , THF or MeCN was used as solvent, and whether the cyclization was performed at room temperature or under reflux. 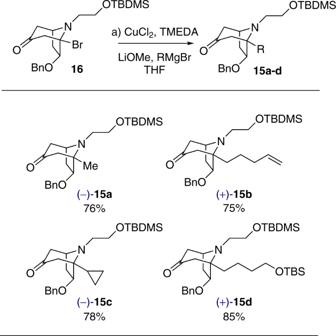Fig. 4: Direct alkylation of 16 with Grignard reagents. Reagents and conditions:aCuCl2, TMEDA, LiOMe, RMgBr, THF, rt, 30 min. Running the reaction in the presence of a base (NEt 3 , DBU, NaOEt, or NaH) led to the formation of a mixture of 7 – 9 (see Supplementary Table 4 ). Interestingly, exposing 7 to I 2 /NaHCO 3 in THF at room temperature produced the unexpected iodoetherification product 31 as a single diastereomer in 86% yield (Fig. 7b ). A plausible mechanism for the diastereoselective formation of 31 is depicted in Fig. 7b [69] . Fig. 7: Attempted transformations of 7–9 into 1. a Reaction of 8 and 9 with TMSCl. b Reaction of 7 with I 2 . Full size image Finally, a dibromination tactic [70] was explored (Fig. 8 ). To avoid possible interference of the hydroxyl group, 7 – 9 were converted to TMS-protected 30 in 95% yield. Compound 30 reacted with Br 2 regioselectively at C11–C12 alkene to afford 32 as a diastereomeric mixture. Unexpectedly, subsequent treatment of this mixture with DBU in CH 2 Cl 2 caused it to revert back to 30 . Finally, we were pleased to find that treating 32 with TBAF in THF yielded stemofoline ( 1 ) directly in 50% yield, isostemofoline ( 2) in 10% yield, and stemoburkilline ( 7 ) in 12% yield. 1 H and 13 C NMR and polarimetric data of stemofoline ( 1 ) {[ α ] D 25 +276 ( c 1.0, MeOH); lit. [25] [ α ] D 25 +273 (MeOH); lit. [28] [ α ] D 25 +270 ( c 0.8, MeOH)}, and isostemofoline ( 2 ) {[ α ] D 25 +102.1 ( c 0.5, CHCl 3 )} were fully consistent with those reported in earlier studies (see Supplementary Tables 11 – 13 ), which confirmed not only the structures including relative and absolute stereochemistries of our synthetic stemofoline ( 1 ) and isostemofoline ( 2 ), but also those of stemoburkilline ( 7 ), (11 S ,12 R )-dihydrostemofoline ( 8 ), and (11 S ,12 S )-dihydrostemofoline ( 9 ). Fig. 8: Completion of the total syntheses of stemofoline (1) and isostemofoline (2). Reagents and conditions: a LHMDS, TMSCl, THF, −78 °C, 1 h, 95%; b Br 2 , CH 2 Cl 2 , rt, 30 min; c TBAF, THF, 0 °C, 1 h, 50% for 1 ; 10% for 2 ; 12% for 7 (for 2 steps from 30 ). Full size image In summary, we have achieved the total synthesis of stemofoline ( 1 ) after it was first isolated and structurally characterized 50 years ago. Our method features a relatively concise (19 steps) route that leads to multiple biomedically relevant compounds in an enantioselective manner. Particularly, we were able to simultaneously obtain stemofoline ( 1 ) and isostemofoline ( 2 ), two other members belonging to the same group stemoburkilline ( 7 ), (11 S ,12 R )-dihydrostemofoline ( 8 ), as well as the (11 S ,12 S )-diastereomer 9 at step 16 of the total synthesis. We argue that our success could be, at least in part, contributed to, and confirm, our biogenetic hypothesis. Furthermore, the synthetic efficiency that we accomplished was also ensured by: (1) an improved three-step protocol that allowed the gram-scale synthesis of keto-lactam cis- 17 , (2) a Cu-catalyzed direct nucleophilic alkylation reaction of 3-bromotropinone 16 , (3) a concise eight-step route for the efficient and selective construction of the pentacyclic core 12 , (4) the successful use of Horner–Wadsworth–Emmons reaction to assemble the two segments of the target molecules, and (5) the convergent transformation of 7 – 9 via 30 to biomimetically forge stemofoline ( 1 ) and isostemofoline ( 2 ). The realization of this bioinspired approach allowed us to predict that (11 S ,12 S )-dihydrostemofoline ( 9 ) might be a natural product yet to be discovered. 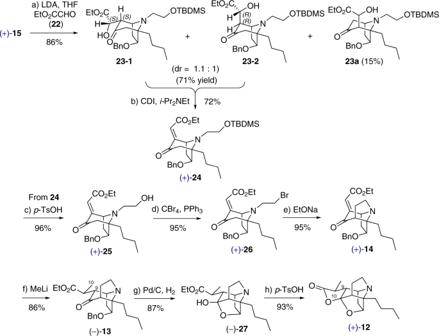Fig. 5: Synthesis of the pentacyclic lactone 12. Reagents and conditions:aLDA, ethyl glyoxalate (22), −78 °C, 1.5 h, 71% for23and 15% for23a; (b) CDI,i-Pr2NEt, DMAP, CH2Cl2, 0 °C to rt, 4 h, 72%;cp-TsOH, acetone, 50 °C, 30 min, 96%;dCBr4, PPh3, CH2Cl2, 0 °C, 30 min, 95%;eEtONa, THF, 0 °C, 20 min, 95%;fMeLi, DMPU, Et2O, −40 °C, 20 min, 86%;gPd/C, H2, EtOH, rt, 2 d, 87%;hp-TsOH, toluene, 85 °C, 2 h, 93% (83% for two steps from13without further purification). The direct, flexible, and versatile introduction of different side chains at C3 of 16 to form 15a – 15d opened an avenue for the synthesis of other stemofoline alkaloids such as methylstemofoline ( 6 ) and its analogues. Moreover, this strategy may also find application in the synthesis of other Stemona alkaloids. General All reactions were performed anhydrously under nitrogen atmosphere. All reagents were purchased from commercial suppliers without further purification. Solvent purification was conducted according to Purification of Laboratory Chemicals (Peerrin, D.D. ; Armarego, W.L. and Perrins, D.R., Pergamon Press: Oxford, 1980). Yields were calculated based on the weights of chromatographically isolated products. Reactions were monitored by thin-layer chromatography (TLC) on plates (GF254) supplied by Yantai Chemicals (China). The TLC spots were visualized under ultraviolet light or by staining with an ethanolic solution of phosphomolybdic acid and cerium sulfate or iodine vapor. Flash column chromatography was performed using silica gel (200–300 mesh) from Qingdao Haiyang Chemicals. NMR spectra were recorded on Bruker AV III 400, Bruker AV III 500, Bruker AV III 850 instruments, and calibrated with tetramethylsilane (TMS) ( δ H = 0.00 ppm) and CDCl 3 ( δ C = 77.00 ppm) as internal references. Multiplicities were designated as follows: s = singlet, d = doublet, t = triplet, q = quartet, br = broad, dd = double doublet, td = triple doublet, dt = double triplet, dq = double quartet, m = multiplet. Infrared spectra were measured on a Nicolet FT-380 spectrometer using film KBr pellet techniques. High-resolution mass spectra analyses were performed on a Fourier transform ion cyclotron resonance mass spectrometer (Bruker Daltonics) with a 7-T magnet (Magnex) and an electrospray ionization source (Apollo II, Bruker Daltonics) under positive-ion mode. Optical rotations were measured on an Anton Paar MCP-500 polarimeter. Experimental data For detailed experimental procedures, see Supplementary Methods. 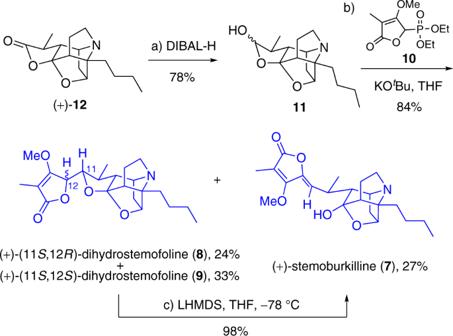Fig. 6: Completion of the total syntheses of stemoburkilline (7), (11S,12R)-dihydrostemofoline (8), and (11S,12S)-dihydrostemofoline (9). Reagents and conditions:aDIBAL-H, CH2Cl2, −78 °C, 30 min, 78%;bt-BuOK,10, THF, 0 °C, 30 min, 84% (27% for7; 24% for8; 33% for9);cLHDMS, THF, −78 °C, 1 h, 98%. NMR spectra were presented as Supplementary Figs. 11 – 66 . For NMR comparison between the reference compounds and compounds that we synthetized in this study, including stemofoline ( 1 ), isostemofoline ( 2 ), stemoburkilline ( 7 ) and (11 S ,12 R )-dihydrostemofoline ( 8 ), see Supplementary Tables 5 – 13 . 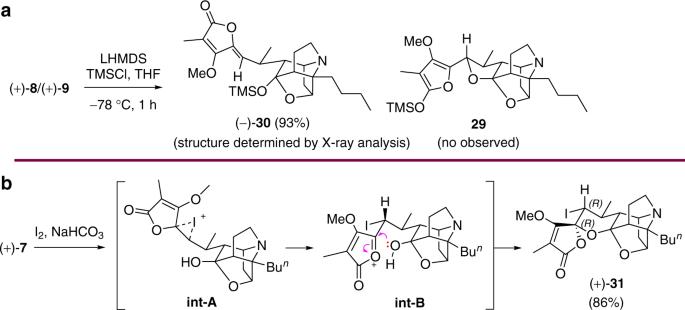Fig. 7: Attempted transformations of 7–9 into 1. aReaction of8and9with TMSCl.bReaction of7with I2. 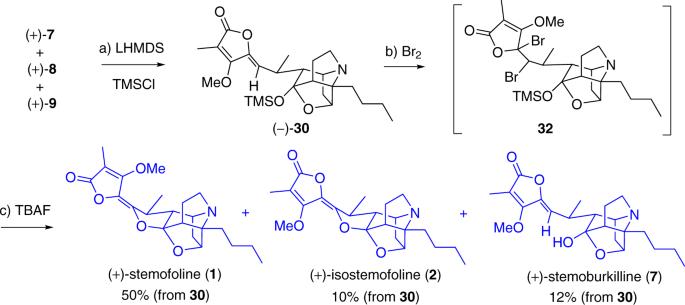Fig. 8: Completion of the total syntheses of stemofoline (1) and isostemofoline (2). Reagents and conditions:aLHMDS, TMSCl, THF, −78 °C, 1 h, 95%;bBr2, CH2Cl2, rt, 30 min;cTBAF, THF, 0 °C, 1 h, 50% for1; 10% for2; 12% for7(for 2 steps from30). For ORTEP diagrams for compounds 30 , see Supplementary Fig. 13 .